Negative Poisson’s ratios in metal nanoplates The Poisson’s ratio is a fundamental measure of the elastic-deformation behaviour of materials. Although negative Poisson’s ratios are theoretically possible, they were believed to be rare in nature. In particular, while some studies have focused on finding or producing materials with a negative Poisson’s ratio in bulk form, there has been no such study for nanoscale materials. Here we provide numerical and theoretical evidence that negative Poisson’s ratios are found in several nanoscale metal plates under finite strains. Furthermore, under the same conditions of crystal orientation and loading direction, materials with a positive Poisson’s ratio in bulk form can display a negative Poisson’s ratio when the material’s thickness approaches the nanometer scale. We show that this behaviour originates from a unique surface effect that induces a finite compressive stress inside the nanoplates, and from a phase transformation that causes the Poisson’s ratio to depend strongly on the amount of stretch. When stretched, materials with a negative Poisson’s ratio become thicker in the direction perpendicular to the original force [1] , [2] , [3] , [4] , [5] , [6] , [7] , [8] , [9] , [10] , [11] . Materials exhibiting such counterintuitive behaviour, known as auxetics, are of great interest not only because they are rare, but also because of their numerous potential applications in various fields, such as the design of fasteners [12] , prostheses [13] , pizeocomposites [14] , [15] , filters [16] , earphones [17] , seat cushions [18] , [19] and superior dampers [20] . Materials with negative Poisson’s ratios have been extensively studied since Lakes [1] reported a negative Poisson’s ratio in a reentrant foam structure. Reentrant foam structure is an example of ‘structural networks’ [2] , [3] , [4] , [5] , [21] , [22] , [23] that manifest a negative Poisson’s ratio, whereas their components at the molecular or microscale level have positive Poisson’s ratios. Among structural networks are molecular networks [3] , hierarchical structures [4] , composites [5] and hinged structures [22] , [23] . Some materials exhibit auxetic properties as they are stretched or compressed in a proper direction [6] , [7] , [8] , [9] , [24] , [25] , [26] , [27] , [28] , [29] , [30] . For example, Baughman et al. [7] reported that 69% of all cubic materials exhibit a negative Poisson’s ratio along the [ ]-direction when they are subjected to stretching along the [110]-direction. The origin of such single-crystal directional stretching had been previously explained by Milstein and Huang [9] . Negative Poisson’s ratios were also observed in some materials near phase transitions [31] , [32] , [33] , [34] , [35] . For example, Hirotsu [31] , [32] reported that Poisson’s ratio of polymer gels becomes negative near the critical point of volume–phase transition. During the ferroelastic transition near the Curie point, barium titanate ceramic exhibits a negative Poisson’s ratio as well [35] . In addition, intermediate valent materials, such as samarium sulphide doped properly with lanthanum, yttrium or thulium, can exhibit negative Poisson’s ratios in all directions [36] , [37] . On the other hand, by using theoretical analysis and computer simulations, Wojciechowski [38] , [39] , [40] , [41] showed that a negative Poisson’s ratio can be found in isotropic and thermodynamically stable two-dimensional models of materials, as well as in harmonic and tethered solids in any dimensionality under negative pressure [42] . Norris [43] provided analytic expressions of the extreme values of Poisson’s ratio over all possible directions for cubic materials. Paszkiewicz and Wolski [44] and Brańka et al. [45] , [46] derived a general expression as a function of elastic constants for the anisotropic Poisson’s ratio and conditions for the classification of any cubic material as auxetics, directional auxetics or non-auxetics. Especially, rare-earth alloys being auxetic in all direction and a few metal alloys exhibiting extreme directional auxetic behaviours were reported together with hundreds of non-auxetic materials [45] . However, all known auxetic materials are bulk materials, and to our knowledge there has been no study to systematically search for negative Poisson’s ratio materials at the nanoscale. By virtue of the enhancement of nanotechnology, numerous layered structures with a thickness of several atomic layers have been achieved for various applications, through experimental techniques such as atomic layer deposition, thermal evaporation, chemical vapour deposition and molecular beam epitaxy methods [47] , [48] , [49] . Therefore, a fundamental understanding of the elastic behaviour of nanoscale plate-shaped materials becomes more important. The effects of free surface on the mechanical properties of nanostructures like nanoparticles, nanowires and nanoplates at unstrained state were systematically discussed by Dingreville et al. [50] They incorporated the surface free energy into the continuum theory of mechanics and obtained effective elastic constants of nanostructures. For example, the Poisson’s ratio of the nanowire increases whereas the biaxial Poisson’s ratio of the nanoplate decreases as the thickness of the nanowire or nanoplate decreases. All of Poisson’s ratios they studied were larger than 0.4 and thus they did not address negative Poisson’s ratios in nanostructures. In this study, we show that negative Poisson’s ratio is a feature of several metal plates with the nanometer thickness under finite strain, contrasting to their bulk counterparts that exhibit positive Poisson’s ratios. For this, we investigate a phase transformation under a proper loading condition and a nanoscale surface effect. The phase transformation induced by the intrinsic instability of cubic materials provokes different amounts of deformation along the two lateral directions. In addition, the relaxation of free surface generates a large compressive stress as a function of thickness and results in changing the Poisson’s ratios of the nanoplates. We illustrate that the phase transformation and pronounced surface effect are two essential conditions for the auxetic behaviour of metal nanoplates. Negative Poisson’s ratio in Al (001) nanoplates Using molecular statics (MS) calculations, we have investigated the Poisson’s ratio of a wide range of metal nanoplates, silicon nanoplates and different type of free surfaces. We first present our results for aluminium (Al) (001) nanoplates of different thicknesses under uniaxial loading. For convenience of notation, we assign here the x- , y- and z- directions to the [100]-, [010]- and [001]-directions, which correspond to the loading, in-plane lateral and thickness directions, respectively. As we apply uniaxial loading in the x- direction, there is only one non-zero stress component of S xx , whereas the others are zero ( S yy =S zz =S yz =S zx =S xy =0). See Methods for details. 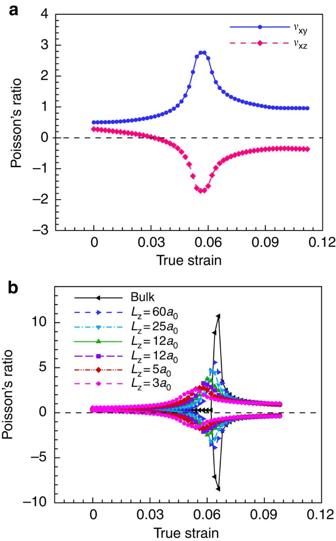Figure 1: Poisson’s ratio of Al (001) nanoplates. (a) The Poisson’s ratio of an Al (001) nanoplate with a thickness of 5a0(2.02 nm) under uniaxial tensile stress along the [100]-direction. (b) The Poisson’s ratio of Al (001) nanoplates with various thicknesses. There is branching for all cases, and the smoothing of the branching becomes more dominant as the thickness decreases. Figure 1a shows the Poisson’s ratio of an Al (001) nanoplate with a thickness of 5 a 0 (where a 0 is the lattice parameter of Al) as a function of applied stretch. Poisson’s ratio is strongly dependent on the amount of stretch and one component ( ν xy ) increases while the other component ( ν xz ) decreases until the strain reaches 5.7%. Along the y- direction, the contraction accelerates as the loading along the x- direction increases to finally reach a Poisson’s ratio of 2.8 at a strain of 5.7%, which signifies that the nanoplate shrinks about three times more along the in-plane lateral direction than it does in the loading direction. Along the z- direction, the Poisson’s ratio initially decreases monotonically and becomes negative at a strain of 3.2%, which signifies that the nanoplate contracts for a while (up to this strain value) and then expands along the thickness direction. It becomes auxetic and this Poisson’s ratio reaches −1.7 at a strain of 5.7%. The Poisson’s ratio becomes less strongly negative as the strain increases further, but it still remains negative even for very large strains (>9%). Figure 1: Poisson’s ratio of Al (001) nanoplates. ( a ) The Poisson’s ratio of an Al (001) nanoplate with a thickness of 5 a 0 (2.02 nm) under uniaxial tensile stress along the [100]-direction. ( b ) The Poisson’s ratio of Al (001) nanoplates with various thicknesses. There is branching for all cases, and the smoothing of the branching becomes more dominant as the thickness decreases. Full size image To study the effect of nanoplate thickness on Poisson’s ratio, we examined Al (001) nanoplates with different thicknesses ranging from 3 a 0 to 60 a 0 ( Fig. 1b ). As the thickness varies, the Poisson’s ratio changes considerably as a function of the applied strain, and also the maximum and minimum Poisson’s ratios vary. For example, the maximum Poisson’s ratio reaches to 4.6 in the in-plane lateral direction and the minimum reaches to −3.2 in the thickness direction, for an Al (001) nanoplate with a thickness of 25 a 0 . In addition, the onset strain at which the Poisson’s ratio in the thickness direction becomes negative changes as well; it increases as the thickness increases. The behaviour of the Poisson’s ratio in bulk material is rather different. In bulk, the Poisson’s ratios in both the thickness and the in-plane lateral directions are equal and positive unlike nanoplates. They are nearly constant until the strain reaches 6%, and they change suddenly for a strain of 6–7% ( Fig. 1b ). The Poisson’s ratio converges to ~1.0 in the in-plane lateral direction and approximately −0.3 in the thickness direction for a large strain (>9%). This branching of the Poisson’s ratios in bulk material is a manifestation of the phase transformation that arises as a result of the instability of materials. As Hill and Milstein [51] , [52] predicted, a material becomes unstable when its elastic stiffness tensor loses its positive definiteness. The general condition for stability is , where B is the elastic stiffness matrix in the Voigt notation. It is equivalent to the condition det[ C ]>0, where C is the elastic moduli matrix, in the case of uniaxial stretch in a principal direction for face-centered cubic (FCC) crystals. For a uniaxial loading in the [100]-direction, this condition reduces further to C 22 – C 23 >0. One can derive the deformation mode for this phase transformation by solving the eigenvalue problem of det[ C –λ I ]=0. The corresponding deformation mode for uniaxial stretch in the [100]-direction is ( δ ε 1 , δ ε 2 , δ ε 3 , δ ε 4 , δ ε 5 , δ ε 6 )=(0, 1,–1, 0, 0, 0) in the Voigt notation, which is a combination of a sudden expansion in one lateral direction and a sudden contraction in the other lateral direction with respect to the loading direction. It is noteworthy that phase transformation accompanies the formation of domains of different phases. Even in a complete transformation from one phase to another in a single crystal, the formation and propagation of domains can be observed. For example, in a molecular dynamics study, the transformation of a metal nanowire from an initial FCC structure to a final face-centered tetragonal structure begins from the formation of face-centered tetragonal domains and terminates by the annihilation of the FCC domain [53] . However, because we employed statics simulations, we have observed a homogeneous deformation as a result of the complete transformation rather than such domain formations in our MS and density functional theory (DFT) calculations, which is consistent with the previous statics studies [54] , [55] , [56] . 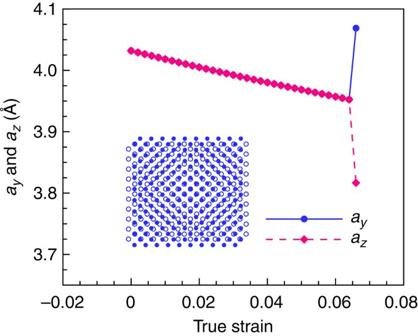Figure 2: Phase transformation for bulk Al (100) under uniaxial loading. Change in the lattice parametersay[010] andaz[001] of bulk Al (100) under uniaxial tensile stress in the [100]-direction is shown. Both lattice parameters reduce equally as the stretch increases, and there is a sudden expansion in they-direction and a sudden contraction in thez-direction at the critical strain of 6.4%. It is the deformation mode of bulk Al (001) that corresponds to the instability conditionC22=C23. The crystal symmetry of the bulk material changes homogeneously from tetragonal to orthorhombic. Atomic positions before (solid dots) and after (open dots) the phase transformation are compared in inset. Figure 2 shows the lattice parameters a y [010] and a z [001] of bulk Al (100) under uniaxial tensile loading in the [100]-direction. As strain is applied to the structure, both lattice parameters reduce gradually and equally, then a sudden deformation happens right after strain 6.4%. In particular, the crystal symmetry of the bulk material under loading in the [100]-direction changes homogeneously from tetragonal to orthorhombic when the condition C 22 = C 23 is satisfied, and this symmetry change explains the branching of the Poisson’s ratios and the occurrence of two different Poisson’s ratios for larger strain (>7%), as shown in Fig. 1b . We note that the branching of the Poisson’s ratio curves in Fig. 1b , for bulk material as well as for nanoplates, originates primarily from the phase transformation. Figure 2: Phase transformation for bulk Al (100) under uniaxial loading. Change in the lattice parameters a y [010] and a z [001] of bulk Al (100) under uniaxial tensile stress in the [100]-direction is shown. Both lattice parameters reduce equally as the stretch increases, and there is a sudden expansion in the y- direction and a sudden contraction in the z- direction at the critical strain of 6.4%. It is the deformation mode of bulk Al (001) that corresponds to the instability condition C 22 = C 23 . The crystal symmetry of the bulk material changes homogeneously from tetragonal to orthorhombic. Atomic positions before (solid dots) and after (open dots) the phase transformation are compared in inset. Full size image Surface effects on Poisson’s ratio As shown in Fig. 1b , the behaviour of nanoplates becomes closer to that of bulk material as the thickness increases, but diverges as the thickness decreases. On the basis of this observation, we conclude that the effect of the phase transformation becomes diluted when the thickness decreases. In other words, the surface effect of nanoplates becomes more dominant as the plates become thinner, resulting in a smoothing of the branching of the Poisson’s ratio. To examine this smoothing tendency in nanoplates relative to their bulk counterpart, we compare the stress distribution along the in-plane lateral direction and the thickness direction ( Fig. 3a ). Note that the total stresses in the two directions are zero as we apply uniaxial loading in the x- direction only. However, the stress inside the nanoplate in the y- direction is non-zero. The stress is very high and tensile on the first layer, and moderate and compressive on the next few layers from the (100) free surfaces. The stresses on the other layers are nearly constant and compressive, so as to compensate for the high tensile stress on the free surface. As a result, the stress field in the nanoplates along the in-plane lateral direction is not homogeneous, unlike in bulk. This is a unique characteristic of nanoplates and is ascribable to the so-called surface effect. The amount of compressive stress is determined by the tensile stress on the free surface of a nanoplate and the number of layers within it, because the total sum of the stresses on the entire nanoplate should be zero. Therefore, the amount of compressive stress increases as the thickness decreases ( Fig. 3b ), and it is inversely proportional ( S~ 1 t −1 ) to the thickness of (001) nanoplates ( Fig. 3c ). Owing to the existence of the (001) free surface, the atoms inside nanoplates are under the tensile stress in the loading direction as well as under the compressive stress in the in-plane lateral direction for finite strains. As a result, the crystal symmetry of inside the Al (001) nanoplates is no longer tetragonal for finite strain. That is why the (001) nanoplates have two different Poisson’s ratio values, whereas the bulk counterpart maintains its tetragonal symmetry and has one single Poisson’s ratio value before the branching. 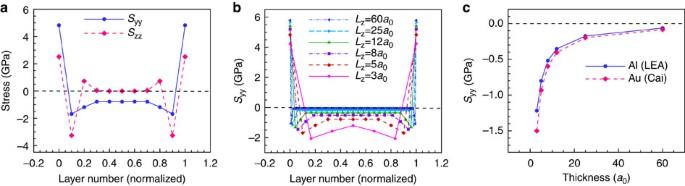Figure 3: Stress distribution of Al (001) nanoplates and stress versus thickness. (a) Stress profile of a 2-nm-thick Al (001) nanoplate throughout its thickness at a strain of 1.0%. The stresses along thez-direction are zero for the layers inside the nanoplate, whereas the stresses along they-direction are not. (b) Stress profiles of Al (001) nanoplates with different thicknesses at a strain of 1.0%. For all cases, stresses along they-direction inside nanoplates are compressive, and they increase as the thickness decreases. (c) Relationship between compressive stress and the thickness of Al and Au (001) nanoplates. The compressive stress is inversely proportional to the thickness for all seven FCC metal (001) nanoplates we considered. Figure 3: Stress distribution of Al (001) nanoplates and stress versus thickness. ( a ) Stress profile of a 2-nm-thick Al (001) nanoplate throughout its thickness at a strain of 1.0%. The stresses along the z -direction are zero for the layers inside the nanoplate, whereas the stresses along the y- direction are not. ( b ) Stress profiles of Al (001) nanoplates with different thicknesses at a strain of 1.0%. For all cases, stresses along the y- direction inside nanoplates are compressive, and they increase as the thickness decreases. ( c ) Relationship between compressive stress and the thickness of Al and Au (001) nanoplates. The compressive stress is inversely proportional to the thickness for all seven FCC metal (001) nanoplates we considered. Full size image So far, we have discussed the existence of compressive stress in the in-plane direction as a consequence of the free surface in the nanoplates. The question that arises next is what effect does this compressive stress have on the Poisson’s ratios? To answer to this question, we intentionally assign compressive stresses in the in-plane lateral direction for bulk Al (001), and then repeat simulations. We apply periodic boundary conditions in all directions, thereby imposing no free surface. Under the assigned compressive stress ( S yy ) in the y -direction, we determine the deformation that makes the stress ( S zz ) in the z -direction zero. The results in terms of Poisson’s ratio are plotted in Fig. 4a for different values of S yy . Poisson’s ratio changes drastically as the stretch increases. Larger compressive stress induces larger changes in the Poisson’s ratios until they reach the extrema. 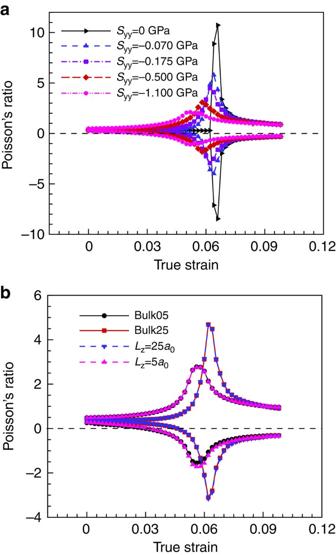Figure 4: Effect of compressive stress on Poisson’s ratio. (a) Poisson’s ratio of bulk Al (001) for assigned compressive stresses along they-direction. Larger compressive stress induces a larger change before reaching extreme points (<5.2%), and a smaller change beyond the extreme points (>5.2%). (b) Comparison of bulk Al (001) under the assigned compressive stress to natural Al (001) nanoplates. The same amount of the compressive stress induced inside each nanoplate is assigned to the corresponding bulk model for comparison. Figure 4: Effect of compressive stress on Poisson’s ratio. ( a ) Poisson’s ratio of bulk Al (001) for assigned compressive stresses along the y- direction. Larger compressive stress induces a larger change before reaching extreme points (<5.2%), and a smaller change beyond the extreme points (>5.2%). ( b ) Comparison of bulk Al (001) under the assigned compressive stress to natural Al (001) nanoplates. The same amount of the compressive stress induced inside each nanoplate is assigned to the corresponding bulk model for comparison. Full size image In Fig. 4b , we show the results from two different material models: a bulk material and a nanoplate. The same amount of the compressive stress induced inside each nanoplate is assigned to the corresponding bulk model for comparison. Remarkably, the outputs of the two models are very similar to one another, indicating that the compressive stress in the in-plane lateral direction plays an important role in inducing a negative Poisson’s ratio as well as causing drastic changes in the Poisson’s ratio as a function of stretch. Different compressive stresses arising from different thicknesses are responsible for the different smoothing of the branching in the Poisson’s ratios. Poisson’s ratios in other cubic (001) nanoplates In Fig. 5a , we compare the changes in Poisson’s ratio of FCC (001) nanoplates of seven metals such as Al, Ni, Cu, Pd, Ag, Pt and Au. Here we model all nanoplates with a uniform thickness of 5 a 0 , and employ a different interatomic potential in the description of the interaction between metal atoms to exclude any artificial effect that may arise from the usage of a single potential. All FCC (001) nanoplates we considered to exhibit the same phenomena—that is, a negative Poisson’s ratio in the thickness direction, and a relatively large positive Poisson’s ratio in the in-plane lateral direction for finite strains. Although there are a little bit different values of Poisson’s ratio resulting from different induced-compressive stresses for employed elements, Poisson’s ratios in the thickness direction of all FCC (001) nanoplates turn to be negative at finite strain (>3.0%). The change in Poisson’s ratios is the largest in Cu nanoplate and the smallest in Au nanoplate. 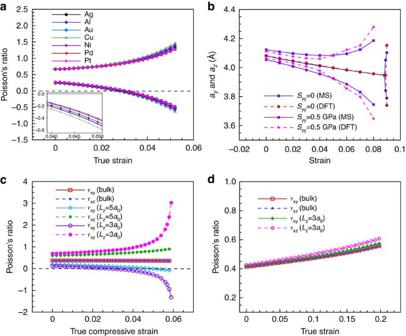Figure 5: Compasion of Poisson’s ratio among different cubic nanoplates. (a) Poisson’s ratio of seven FCC (001) nanoplates each with a thickness of 5a0. All nanoplates exhibit the same behaviour: a negative Poisson’s ratio in the thickness direction and a relatively large positive Poisson’s ratio in the in-plane lateral direction at finite strain (>3.0%). (b) Comparison of DFT and MS results in the effect of compressive stress. Under assigned compressive stresses in the in-plane lateral (y-) direction, the changes in the lattice parameters of bulk Au (001) under loading in thex-direction are shown. (c) Poisson’s ratio of Fe (001) nanoplates with thickness of 3a0and 5a0as examples of BCC metals. Fe (001) nanoplate shows the same behaviour as FCC (001) nanoplates. (d) Poisson’s ratio of a Si (001) nanoplate with a thickness of 3a0. Si (001) nanoplates do not exhibit a negative Poisson’s ratio or a drastic change in the Poisson’s ratio, because the tensile stress on the free surface is too small to induce sufficient compressive stresses inside the Si (001) nanoplates. Figure 5: Compasion of Poisson’s ratio among different cubic nanoplates. ( a ) Poisson’s ratio of seven FCC (001) nanoplates each with a thickness of 5 a 0 . All nanoplates exhibit the same behaviour: a negative Poisson’s ratio in the thickness direction and a relatively large positive Poisson’s ratio in the in-plane lateral direction at finite strain (>3.0%). ( b ) Comparison of DFT and MS results in the effect of compressive stress. Under assigned compressive stresses in the in-plane lateral ( y- ) direction, the changes in the lattice parameters of bulk Au (001) under loading in the x- direction are shown. ( c ) Poisson’s ratio of Fe (001) nanoplates with thickness of 3 a 0 and 5 a 0 as examples of BCC metals. Fe (001) nanoplate shows the same behaviour as FCC (001) nanoplates. ( d ) Poisson’s ratio of a Si (001) nanoplate with a thickness of 3 a 0 . Si (001) nanoplates do not exhibit a negative Poisson’s ratio or a drastic change in the Poisson’s ratio, because the tensile stress on the free surface is too small to induce sufficient compressive stresses inside the Si (001) nanoplates. Full size image To underline the generality of our finding and thus enhance the accuracy of our computations, we have performed DFT calculations as well. Because of expensive computational cost, we adopt DFT calculations to one bulk FCC material only. This time, we choose Au instead of Al to confirm the generality of our finding. The comparison of different methods is shown in Fig. 5b . When a uniaxial stress in the loading direction is applied ( S yy =0), two results from DFT and MS models are in excellent agreement. The reductions of the lattice parameters with applied strain are the same in both models. In addition, the critical strain for the phase transformation is 8.8% in MS calculation and it is 8.9% in DFT calculation. When a finite compressive stress ( S yy =0.5 GPa) is applied, the change in the lattice parameters in the DFT calculation is a little bit different from that in the MS calculation. However, a negative Poisson’s ratio in the thickness ( z- ) direction and a drastic change of Poisson’s ratio in the in-plane lateral ( y- ) direction at finite strains are clearly shown in both calculations. In addition, we find that body-centered cubic (BCC) (001) metal nanoplates also exhibit the same phenomena as shown in Fig. 5c . As examples of BCC metals, we model iron (Fe) nanoplates with thickness of 3 a 0 and 5 a 0 . The Poisson’s ratio in the thickness direction of the Fe (001) nanoplate with a thickness of 3 a 0 becomes negative at a strain of ~2.9%, whereas bulk Fe (001) never shows a negative Poisson’s ratio. It is noteworthy that for BCC metals a uniaxial compressive stress, rather than a tensile stress, must be applied to satisfy the condition C 22 = C 23 for a phase transformation. Furthermore, FCC and BCC metal nanoplates show the same behaviour in spite of their contrasting atomic bonding characteristics and different amount of surface relaxation. The change in Poisson’s ratio of silicon (Si) (001) nanoplates with strain is illustrated in Fig. 5d . The Poisson’s ratios of the Si (001) nanoplate with a thickness of 3 a 0 change a little bit as uniaxial loading applied, but they are always positive. Although bulk Si (001) has the same cubic symmetry as FCC and BCC metals, and thus undergoes a definite phase transformation under the uniaxial stretch in the [100]-direction, Si nanoplates do not exhibit the same drastic change in Poisson’s ratio. The (001) free surface plays an important role in changing the Poisson’s ratios of FCC and BCC metals but it does not in those of Si. As shown in Fig. 5d , the Si nanoplate does not exhibit large changes in Poisson’s ratios even though Si (001) bulk has the same cubic symmetry with FCC and BCC metals. To explain this phenomenon, we compare stress profiles in the in-plane lateral direction inside Al, Fe and Si (001) nanoplates throughout their thickness in Fig. 6a . The internal compressive stresses induced by (001) free surfaces are different from one another. The compressive stress inside the Si (001) nanoplates is only ~70 MPa; that is, one order of magnitude lower than that of the inside FCC or BCC nanoplates. The tensile stress on Si (001) free surface is too small to induce a sufficient amount of compressive stresses inside the nanoplates. Consequently, Poisson’s ratios of even a thin Si (001) nanoplate do not change much from that of Si (001) bulk. It is noteworthy that Si (001) nanoplates also exhibit a negative Poisson’s ratio when we intentionally applied a large compressive stress (>1 GPa) in the in-plane lateral direction. 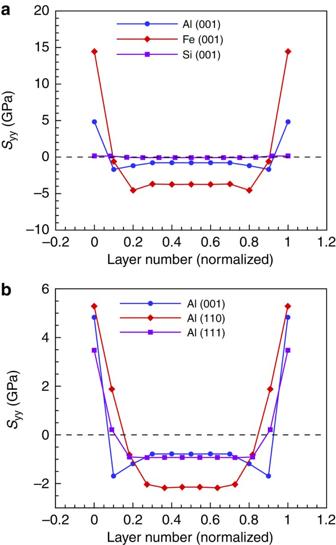Figure 6: Stress profiles in cubic nanoplates with different elements and surfaces. (a) Comparison of the stress profiles in the in-plane lateral direction inside Al, Fe and Si (001) nanoplates. The amount of compressive stress inside Si (001) nanoplates is much lower than that inside FCC or BCC metal nanoplates, and thus it cannot induce negative Poisson’s ratio or a drastic change in Poisson’s ratios. (b) Comparison of the stress profiles of Al nanoplates in the in-plane lateral direction with different free surfaces throughout their thickness. Although the (110) or (111) free surface exhibits high tensile stress on the first layer and thus induces finite compressive stresses in the in-plane lateral direction inside nanoplates, the Poisson’s ratios of the (110) or (111) nanoplates never become negative. Figure 6: Stress profiles in cubic nanoplates with different elements and surfaces. ( a ) Comparison of the stress profiles in the in-plane lateral direction inside Al, Fe and Si (001) nanoplates. The amount of compressive stress inside Si (001) nanoplates is much lower than that inside FCC or BCC metal nanoplates, and thus it cannot induce negative Poisson’s ratio or a drastic change in Poisson’s ratios. ( b ) Comparison of the stress profiles of Al nanoplates in the in-plane lateral direction with different free surfaces throughout their thickness. Although the (110) or (111) free surface exhibits high tensile stress on the first layer and thus induces finite compressive stresses in the in-plane lateral direction inside nanoplates, the Poisson’s ratios of the (110) or (111) nanoplates never become negative. Full size image Comparison with other free surfaces Now, we examine the Poisson’s ratios of metal nanoplates with different free surfaces such as (111) and (110). In Fig. 6b , we compare the stress profiles in the in-plane lateral direction inside Al (001), Al (111) and Al (110) nanoplates with 11 atomic layers in thickness. Like (001) surface, other free surfaces induce finite compressive stresses, and their values are approximately 780 MPa, 920 MPa and 2,140 MPa in order of (001), (111) and (110) nanoplates, respectively. However, as shown in Fig. 7 , the nanoplate with (111) or (110) free surfaces never exhibits a negative Poisson’s ratio, even though the induced-compressive stresses cause large changes in the values of Poisson’s ratios. That is because there is no definite phase transformation in (111) or (110) nanoplates unlike (001) nanoplates. It is noteworthy that the nanoplates considered here are still in elastic range in spite of large stress and strain, because defect-free nanomaterials can support much larger elastic ranges of stress and strain as compared with their bulk counterparts [57] , [58] , [59] . 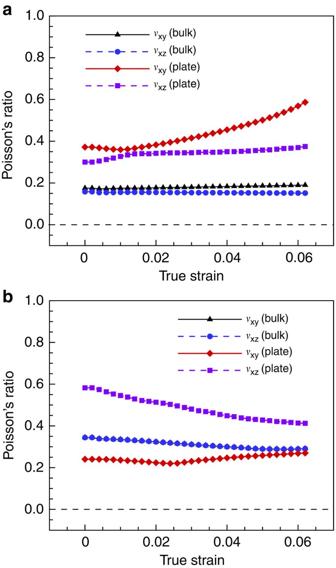Figure 7: Poisson’s ratio of Al (111) and (110) nanoplates. (a) Poisson’s ratio of a 2.79-nm-thick Al (111) nanoplate under uniaxial tensile stress in the []-direction. The compressive stresses inside the nanoplates owing to the (111) free surface make a significant difference to the Poisson’s ratio values, but there is no negative Poisson’s ratio. (b) Poisson’s ratio of a 1.71-nm-thick Al (110) nanoplate under uniaxial tensile stress in the [001]-direction. Again, large compressive stress inside nanoplates owing to the (110) free surface causes different behaviours of the Poisson’s ratio, but it does not reach a negative value. Figure 7: Poisson’s ratio of Al (111) and (110) nanoplates. ( a ) Poisson’s ratio of a 2.79-nm-thick Al (111) nanoplate under uniaxial tensile stress in the [ ]-direction. The compressive stresses inside the nanoplates owing to the (111) free surface make a significant difference to the Poisson’s ratio values, but there is no negative Poisson’s ratio. ( b ) Poisson’s ratio of a 1.71-nm-thick Al (110) nanoplate under uniaxial tensile stress in the [001]-direction. Again, large compressive stress inside nanoplates owing to the (110) free surface causes different behaviours of the Poisson’s ratio, but it does not reach a negative value. Full size image In addition, it is interesting that the compressive stress induced by the (001) free surface produces a negative Poisson’s ratio along the [001]-direction but it reduces a negative Poisson’s ratios along the [ ]-direction. It was reported that 69% of the cubic metals have negative Poisson's ratio along the [ ]-direction, when they are stretched along the [110]-direction [7] , [9] . To underline the effect of (001) free surface, we calculate the Poisson's ratios of six FCC metal nanoplates and their bulk counterpart under the same conditions with the previous reports. All bulk FCC metals we considered show negative Poisson's ratios along the [ ]-direction. However, these negative Poisson's ratios are reduced (Cu and Ni) or even removed (Au, Ag, Pt and Pd) when we introduce the (001) free surface at nanoscale, as shown in Table 1 . Table 1 Comparison of Poisson’s ratios in FCC (001) nanoplates and bulk in the unstrained state. Full size table We have shown that FCC (001) and BCC (001) nanoplates exhibit the negative Poisson’s ratio as they are stretched (FCC) or contracted (BCC). Although Si (001) bulk has the same cubic symmetry with FCC and BCC metals and thus has the definite phase transformation under the uniaxial stretch in the [100] direction, Si nanoplates do not show the drastic change in Poisson’s ratios because the surface effect is not sufficient. On the other hand, tensile stresses at surfaces of the (111) or (110) nanoplates are large enough to cause compressive stress inside the nanoplates, (111) or (110) nanoplates do not exhibit a negative Poisson’s ratio, because they do not have a definite phase transformation under uniaxial stretch. Therefore, both the proper direction of the loading relative to the lattice (needed to cause the Poisson’s ratio branching) and the large surface relaxation (needed to induce sufficient compressive stresses inside nanoplates for the smoothing) are two essential conditions for the creation of a negative Poisson’s ratio. Both of FCC and BCC (001) nanoplates inherently satisfy these conditions. We have found that several metal nanoplates that have (001) free surface and nanoscale thickness exhibit a negative Poisson’s ratio along the thickness directions as they are under uniaxial loading in the [100] direction. As two primary origins for this unveiled behaviour of the metal nanoplates, we have discussed the finite compressive stresses inside the metal nanoplates inherently generated because of the (001) free surface and phase transformation induced by the intrinsic instability of cubic materials. This study reveals another interesting material property of nanostructures, negative Poisson’s ratio, and contributes to the database of auxetic materials that were believed to be uncommon in nature. MS simulation For metal (001) nanoplates, we designate the [100], [010] and [001] directions as x- , y- and z- directions, corresponding to the loading, in-plane lateral and thickness directions, respectively. We apply periodic boundary conditions to the x- and y- directions to model the nanoplates, and to all directions to model the bulk counterpart materials. The size of the nanoplates in the x- and y- directions is 10 a 0 × 10 a 0 , where a 0 is the lattice parameter of the considered element. We have confirmed that larger models give very similar results. We vary the thickness of the nanoplates from 3 a 0 to 60 a 0 . The interaction between Al atoms is described by the interatomic potential developed by Liu et al. [60] , which has been shown to yield excellent results for surface energies and stacking-fault energies under various deformations. For other FCC metal atoms, we employ the interatomic potential proposed by Cai and Ye [61] to exclude any artificial effect that may arise from the usage of a single potential. In the study of a BCC nanoplate, iron atoms are described by another empirical potential [62] . For Si (001) nanoplates, we use the Tersoff potential [63] . Under the MS calculations, all models are fully relaxed to attain the equilibrium state before applying uniaxial loading, and then strain is applied in the x- direction with an increment of 0.1%. To achieve the uniaxial stress condition, the nanoplates are allowed to expand or contract in the y- direction to make the stress in the y- direction zero. The definition of Poisson’s ratios under loading along the x- direction, for infinitesimal strain as well as finite strain, is given by In the numerical evaluation, we use the central finite difference method with second-order accuracy to approximate the Poisson's ratio in equation (1). Then, the Poisson's ratios of a plate at the strain can be obtained using DFT simulation The local density approximation [64] and ultra-soft pseudo-potential [65] are used. We employ 13 × 13 × 13 Monkhorst-Pack [66] meshes for sampling the Brillouin zone. All calculations are relaxed until forces on each ion become less than 0.01 eV Å −1 with a cutoff energy of 400 eV. We utilize the Cambridge Serial Total Energy Package (CASTEP) [67] for DFT calculations. How to cite this article: Ho, D. T. et al. Negative Poisson’s ratios in metal nanoplates. Nat. Commun. 5:3255 doi: 10.1038/ncomms4255 (2014).